Mechanisms of molecular transport through the urea channel ofHelicobacter pylori Helicobacter pylori survival in acidic environments relies on cytoplasmic hydrolysis of gastric urea into ammonia and carbon dioxide, which buffer the pathogen’s periplasm. Urea uptake is greatly enhanced and regulated by Hp UreI, a proton-gated inner membrane channel protein essential for gastric survival of H. pylori . The crystal structure of Hp UreI describes a static snapshot of the channel with two constriction sites near the center of the bilayer that are too narrow to allow passage of urea or even water. Here we describe the urea transport mechanism at atomic resolution, revealed by unrestrained microsecond equilibrium molecular dynamics simulations of the hexameric channel assembly. Two consecutive constrictions open to allow conduction of urea, which is guided through the channel by interplay between conserved residues that determine proton rejection and solute selectivity. Remarkably, Hp UreI conducts water at rates equivalent to aquaporins, which might be essential for efficient transport of urea at small concentration gradients. Chronic gastric infection with Helicobacter pylori affects ~50% of the global population and is the leading cause for peptic ulcer disease and stomach cancer [1] . Survival of H. pylori in acidic environments as low as pH 1 is contingent on the expression of an inner membrane urea channel, Hp UreI [2] . This channel funnels gastric urea to the cytoplasmic urease, where it is hydrolysed into CO 2 and 2NH 3 , which in turn buffer the pathogen’s periplasm to pH 6.1 ( Supplementary Fig. S1 ) [3] . Hp UreI is a urea-selective member of the AmiS/UreI urea-amide channel superfamily [4] . The recently determined crystal structure of Hp UreI (PDB code: 3UX4) showed a hexameric ring of channel protomers [5] . Each protomer consists of a bundle of six transmembrane helices that are arranged around a central channel with three-fold pseudo symmetry relating three pairs of transmembrane helices. The pore is lined by conserved amino-acid side chains that identify the solute pathway for this superfamily [5] . This structure, which is the result of a non-inverted gene triplication, is functionally homologous but structurally and mechanistically completely unrelated to urea transporters (UTs), which are technically also channel proteins and result from an inverted gene duplication [6] , [7] . Furthermore, while Hp UreI and some aquaporins (several of which also conduct urea) are pH gated, UTs generally do not show pH dependency. The structure of Hp UreI revealed a novel pH-gated urea channel architecture. However, the mechanism of urea transport and solute selectivity remained unknown. This is because the crystal structure of the channel, determined at pH 5.3, 0.6 pH units below the pK of opening, showed two constrictions at the center of the bilayer that were too narrow for passage of urea or water, raising the question how the channel manages to conduct and select for urea-like molecules, while excluding protons from the gastric juice, which is essential for the survival of H. pylori . To investigate the mechanism of conduction and selectivity, we have carried out atomic resolution molecular dynamics simulations on the basis of the crystal structure in its biologically active hexameric form. Unlike molecular simulation studies of urea transporter (UT) channels [7] , which applied improved sampling techniques to evaluate the trans-pore-free energy profiles, we present here an alternative approach that captures conduction events from unbiased long-timescale equilibrium molecular dynamics simulations. We show that microsecond simulations of the hexamer were able to capture spontaneous urea permeation events through the protomer channels identified in the crystal structure, confirming that the channels conduct urea ( Fig. 1 ). Guided by this unbiased hexamer simulation, a restrained protomer channel system was constructed that allowed an increase in simulation time to 7 μs, which captured 10 spontaneous conduction events. In addition to equilibrium trans-pore free energy profiles, this approach also provides transport kinetics, as well as the atomic resolution mechanistic details of urea conduction without bias. Simulations of mutants provide further mechanistic insights into the function of the channel. 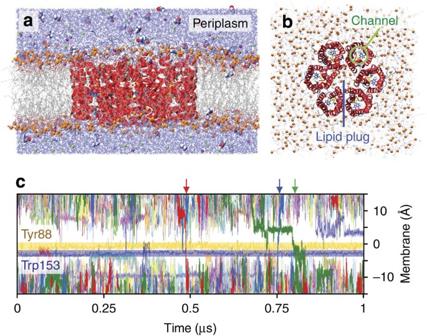Figure 1: Simulation of urea conduction through theHpUreI hexamer. (a) Side view ofHpUreI hexamer in a POPC lipid bilayer in the presence of 150 mM urea and 100 mM NaCl. (b) View from the periplasmic side shows the six channel pores surrounding a central lipid plug containing nine cytoplasmic and three periplasmic lipids. (c) Unrestrained microsecond atomic detail molecular dynamics simulations are able to capture multiple spontaneous transport events (indicated by arrows), showing that transport is a rare event (one urea per hexamer every ~330 ns in the presence of 150 mM urea). The scarcity of urea in the pore illustrates the low urea affinity of the channel. Figure 1: Simulation of urea conduction through the Hp UreI hexamer. ( a ) Side view of Hp UreI hexamer in a POPC lipid bilayer in the presence of 150 mM urea and 100 mM NaCl. ( b ) View from the periplasmic side shows the six channel pores surrounding a central lipid plug containing nine cytoplasmic and three periplasmic lipids. ( c ) Unrestrained microsecond atomic detail molecular dynamics simulations are able to capture multiple spontaneous transport events (indicated by arrows), showing that transport is a rare event (one urea per hexamer every ~330 ns in the presence of 150 mM urea). The scarcity of urea in the pore illustrates the low urea affinity of the channel. Full size image System setup and oligomeric state The crystal structure did not show density for periplasmic loop 1 (PL1), possibly because of the fact that the 6-histidine tag had to be inserted into this loop because N- and C-terminally tagged protein was not active [5] . This 14-residue (without tag) loop was modelled and allowed to equilibrate during a 400 ns simulation of a restrained single protomer in a 92 palmitoyloleoyl-phosphocholine (POPC) lipid bilayer (see Methods). To construct a complete Hp UreI hexamer, the loop was copied and transposed onto the other protomers. The complete hexamer was then embedded into a 370 POPC lipid bilayer and equilibrated at 37 °C in the presence of 100 mM sodium chloride and 150 mM urea, which is below the half-saturation concentration (~163 mM) of the channel [8] , while restraining the protein backbone to the crystal structure. The total system size of the hexamer was ~110,000 atoms (see Fig. 1 and Supplementary Movie 1 ). A complete list of simulation systems is given in Supplementary Table S1 . Knowledge of the oligomeric state of Hp UreI in the membrane is important for understanding how the tetrahedral dodecameric 1.1-MDa complex of the cytoplasmic urease [9] might couple to it [10] . It may also play a role in cooperative pH gating. To investigate the nature of the unusual hexameric ring arrangement, we carried out unrestrained simulations of a single protomer embedded in a lipid bilayer. This resulted in rapid deviation from the native state, ultimately leading to pore collapse within several hundreds of nanoseconds, irrespective of urea concentration ( Supplementary Fig. S2 ). These results were obtained independently with two different force fields (OPLS and CHARMM), suggesting that the hexameric arrangement is essential for maintaining proper helix conformations for each loosely packed protomer and represents the native state in the bilayer. Urea binding affinity Our simulations support experimental observations that Hp UreI has a remarkably low binding affinity for urea [8] . Although urea explores all regions of the channel pore, it only occupies each protomer for ~10% of the total simulation time ( Supplementary Fig. S3 ). This low occupancy is chiefly due to the absence of a high affinity binding site that could form simultaneous hydrogen bonds with the single carbonyl and two amino groups of planar urea. Analysis of the crystal structure revealed that the channel is defined entirely by side chains, 54% of which are hydrophobic. Although approximately half of the side chains lining the channel are able to form hydrogen bonds, urea entry is unfavourable. This is due to the strong polarity of urea. With a liquid state dipole moment of 6–8 Debye (D) [11] (the experimental value for liquid water is 2.95 D [12] , and the value of the TIP3P water model is 2.35 D [13] ), urea has been shown, using ab initio quantum calculations, to attract a first hydration shell of ~6-7 water molecules [14] . Our analysis gives a slightly higher bulk value of 8-9 water molecules in the first hydration shell. Upon entering the Hp UreI channel, urea molecules lose ~3 water molecules from the first hydration shell in the vestibules and ~4 water molecules in the constrictions, which is only partially compensated by hydrogen bonding contacts with channel-lining residues ( Fig. 2 ). A similar compensation mechanism has been observed for aquaporin, bacterial glycerol facilitator, and urea transporter (UT) channels [7] , [15] . However, confinement of the polar urea molecule carries an additional energetic penalty because of the reduction in translational and rotational entropy, which is associated with the strong preferential alignment observed during transport through the pore ( Fig. 2 ). Analysis of the averaged spatial alignment of the urea dipole moment, which is zero in bulk water due to rapid tumbling, revealed a net alignment of up to 5.2 D along most of the transition pathway ( Fig. 2 ). This compares with the theoretical maximum of 8 D for a perfectly immobilized urea molecule. In the channel, urea molecules preferentially orient with their carbonyl group pointing towards the central lipid plug ( Fig. 2 ). 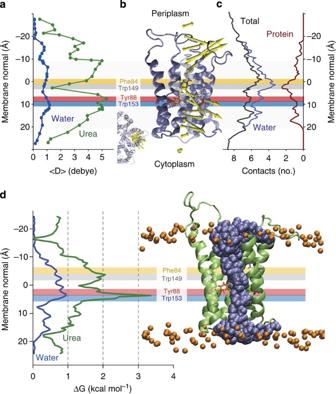Figure 2: Urea transport through theHpUreI channel pore. (a) Magnitude of averaged net urea and water dipole moment along the channel during translocation (system H1, chain F, two events). (b) Urea dipole vectors along the channel pore (chain F). The length of the vector is equivalent to the net strength of the time-averaged dipole moment (the theoretical maximum dipole moments, corresponding to perfectly aligned molecules, are 8 D for urea and 2.4 D for the TIP3P water). Rapid tumbling of urea and water results in net-zero dipole moments in bulk solution. However, inside the pore urea molecules are strongly aligned, with the amino groups pointing away from the central lipid plug. (c) Time-averaged number of contacts of urea with water and protein side chains in the channel. The figure shows that protein side chain contacts cannot fully compensate the loss of water molecules from the hydration shell of urea. (d) Urea transport free energy (ΔG) profile derived from the restrained monomer simulation. The profile shows two main barriers to transport separated by a local free energy minimum. The right panel shows the superposition of the urea carbon atom over the course of the simulation (blue), demonstrating visually that urea fully samples all parts of the channel. Figure 2: Urea transport through the Hp UreI channel pore. ( a ) Magnitude of averaged net urea and water dipole moment along the channel during translocation (system H1, chain F, two events). ( b ) Urea dipole vectors along the channel pore (chain F). The length of the vector is equivalent to the net strength of the time-averaged dipole moment (the theoretical maximum dipole moments, corresponding to perfectly aligned molecules, are 8 D for urea and 2.4 D for the TIP3P water). Rapid tumbling of urea and water results in net-zero dipole moments in bulk solution. However, inside the pore urea molecules are strongly aligned, with the amino groups pointing away from the central lipid plug. ( c ) Time-averaged number of contacts of urea with water and protein side chains in the channel. The figure shows that protein side chain contacts cannot fully compensate the loss of water molecules from the hydration shell of urea. ( d ) Urea transport free energy (ΔG) profile derived from the restrained monomer simulation. The profile shows two main barriers to transport separated by a local free energy minimum. The right panel shows the superposition of the urea carbon atom over the course of the simulation (blue), demonstrating visually that urea fully samples all parts of the channel. Full size image Urea transport rate and channel gating An unrestrained microsecond simulation of the bilayer-embedded Hp UreI hexamer in the presence of 150 mM urea on both sides of the bilayer captured three urea molecules spontaneously permeating through a channel protomer ( Fig. 1 and Supplementary Movie 2 ). Assuming that urea flux is approximately proportional to the concentration of urea below half-saturation this corresponds to a urea transport rate of ~833 s −1 per protomer at urea concentrations of 5 mM, close to the physiological concentration in the gastric juice. This transport rate is within the range of experimental estimates of 200–1,000 s −1 per protomer, derived from urease activity assays in live H. pylori cells [5] . To increase the sampling of the conduction mechanisms and improve the statistical estimate of the conduction rate, we performed two multi-microsecond simulations of single protomers in a lipid bilayer at urea concentrations of 400 mM ( Supplementary Fig. S4 ). To prevent the pore collapse mentioned above, the backbone atoms of the six transmembrane helices were restrained over the entire duration of the simulations. Coordinates were taken from the conducting protomer F at 480 ns (see Supplementary Discussion ). The first simulation showed two conduction events, but after ~300 ns the first periplasmic loop (PL1) was found to fold into the channel vestibule, with residues Asn64, Ile65, Ala66, and Gln67 forming a plug that blocks urea molecules from entering the pore for the remainder of the 2 μs simulation ( Fig. 3 and Supplementary Movie 3 ). Mutation studies have shown that histidine residues on the periplasmic loops are essential for pH gating [16] , suggesting that opening and closing of the channel might be controlled by reversible folding of one or both loops into the periplasmic vestibule of the channel. While the simulation timescales of 2 μs are at least an order of magnitude too short to fully investigate this hypothesis, the results nevertheless show that the PL1 is indeed capable of folding into the periplasmic vestibule of the channel, blocking urea access to the pore in the process. Interestingly, the 1 μs hexamer simulation did not show pore blocking but revealed that residues 55–57 of PL1 generally interact with residues 60–62 of the PL1 of the neighbouring protomer (see Supplementary Fig. S5 ). This suggests that loop folding in the hexamer might be cooperative, explaining why PL1 of a single protomer is unstable and blocks pore access even at pH<5.5, where the majority of channels are open. However, in the absence of an experimental loop structure, the conclusions drawn from the simulations remain speculative. 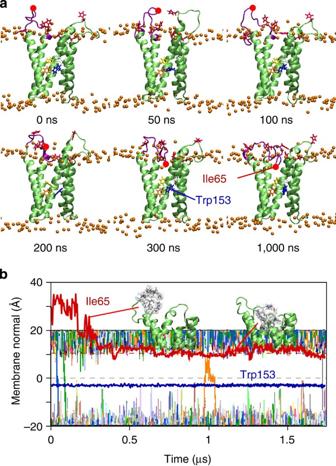Figure 3: Channel closure through periplasmic loop folding. (a) For single-monomer simulations, spontaneous folding of the first periplasmic loop (PL1) into the periplasmic channel vestibule results in pore closure (seeSupplementary Movie 1for details). (b) Position along the membrane normal of a loop residue (Ile65, indicated in red in panela) shows that channel closure is stable for >1.0 μs. Before closure, two spontaneous transport events (blue and green) are observed in the first 200 ns, after which loop folding prevents further urea molecules from entering the periplasmic vestibule. A CCresidue (Trp153, in blue) is shown for reference. Figure 3: Channel closure through periplasmic loop folding. ( a ) For single-monomer simulations, spontaneous folding of the first periplasmic loop (PL1) into the periplasmic channel vestibule results in pore closure (see Supplementary Movie 1 for details). ( b ) Position along the membrane normal of a loop residue (Ile65, indicated in red in panel a ) shows that channel closure is stable for >1.0 μs. Before closure, two spontaneous transport events (blue and green) are observed in the first 200 ns, after which loop folding prevents further urea molecules from entering the periplasmic vestibule. A C C residue (Trp153, in blue) is shown for reference. Full size image To prevent pore closure, a second 7-μs simulation was performed with the loop restrained in an ‘open’ configuration. This simulation captured 10 spontaneous conduction events (see Supplementary Fig. S4 and Supplementary Movie 4 ), corresponding to a uni-directional single-channel transport rate of ~7 × 10 5 s −1 at 400 mM urea (~9 × 10 3 s −1 at 5 mM). Grey et al. reported conduction rates in proteoliposomes of ~500,000 s −1 in the presence of 400 mM urea gradients for Hp UreI [8] . These measurements were performed at pH 5 in Escherichia coli polar lipid vesicles of 100±10 nm diameter, with a per-weight protein-to-lipid ratio of 1/100, which corresponds to ~5-6 Hp UreI hexamers per proteoliposome. Assuming all channels are open and functional, irrespective of their orientation in the vesicular membrane, the equivalent single-channel urea flux rate is ~1.3–1.6 × 10 4 s −1 , an order of magnitude smaller than observed in our simulations. While the rate of urea transport is low for a channel protein, our simulations reveal that a conducting urea molecule takes just 7±5 ns to cross the entire length of the pore (see Supplementary Table S2 ). This is much shorter than the mean time between consecutive permeation events (Δt′=0.7 μs). In contrast, ion channels, which typically have much higher conduction rates, also have much longer dwell times. A recent simulation study found that for voltage-gated sodium channels the dwell time is approximately twice as long as the time between conduction events [17] . Comparison of the motion of channel-lining residues and the atomic detail conduction mechanism showed that the spontaneous transport of urea closely resembled that determined in the hexamer simulation (see Supplementary Discussion and Supplementary Figs S6 and S7 ). Urea conduction mechanism Each protomer in the Hp UreI crystal structure revealed two closely spaced constrictions near the center of the bilayer that obstruct the solute pathway [5] . The first constriction (C P ) in the channel, located at the end of the periplasmic vestibule, is formed by the side chains of the conserved residues Leu6, Val9, Phe84, Trp146, and Trp149. This constriction is very hydrophobic and presumably acts as the proton filter. The second constriction (C C ) is adjacent, located ~7 Å closer towards the cytoplasm. C C is formed by the side chains of conserved residues Val9, Leu13, Trp153, Tyr88, and Glu177. In the crystal structure, both constrictions were found to be too narrow to allow the passage of urea or even water through the channel. The simulations reveal in atomic detail how these constrictions open and allow the passage of urea and water ( Fig. 4 ). 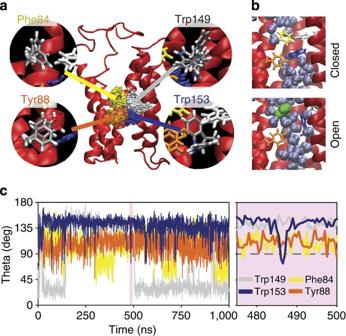Figure 4: Opening and closing of the two constrictions is regulated by the orientation of aromatic rings inside the channel pore. (a) The total configurational space sampled by the key aromatic residues of the periplasmic constriction (CP): Phe84 (yellow) and Trp149 (white), and the cytoplasmic constriction (CC): Tyr88 (orange) and Trp153 (blue). Each aromatic has only a small number of accessible states defined by the angle of its aromatic ring normal with respect to the membrane normal (Supplementary Fig. S20). Representative equilibrium states of the ring orientations are shown in the circular panels. Tyr88 has one state, Phe84 and Trp153 have two states, whereas Trp149 has four. (b) Snapshots of the open and closed constriction. (c) Time evolution of the aromatic ring tilt angle. Rotation of Trp153 from the horizontal (~150°) to the vertical (~80°) orientation switches the channel from a closed to an open state that enables urea conduction at 486 ns (shaded). The opening motion is towards the periplasm, in the direction of the approaching urea. Figure 4: Opening and closing of the two constrictions is regulated by the orientation of aromatic rings inside the channel pore. ( a ) The total configurational space sampled by the key aromatic residues of the periplasmic constriction (C P ): Phe84 (yellow) and Trp149 (white), and the cytoplasmic constriction (C C ): Tyr88 (orange) and Trp153 (blue). Each aromatic has only a small number of accessible states defined by the angle of its aromatic ring normal with respect to the membrane normal ( Supplementary Fig. S20 ). Representative equilibrium states of the ring orientations are shown in the circular panels. Tyr88 has one state, Phe84 and Trp153 have two states, whereas Trp149 has four. ( b ) Snapshots of the open and closed constriction. ( c ) Time evolution of the aromatic ring tilt angle. Rotation of Trp153 from the horizontal (~150°) to the vertical (~80°) orientation switches the channel from a closed to an open state that enables urea conduction at 486 ns (shaded). The opening motion is towards the periplasm, in the direction of the approaching urea. Full size image During the simulations C P opens by outward tilting of helices A, C and F, while helix D tilts inwards. The resulting structural rearrangement permanently widens the channel diameter by ~2 Å at C P , enough to open the constriction for conduction of urea molecules (see Supplementary Figs S8 and S9 ). Control simulations of restrained protomers before opening of C P showed no conduction, suggesting this rearrangement is required for urea to pass through the pore (see Supplementary Discussion and Supplementary Fig. S10 ). During transition through C P , urea was found to be sandwiched between the aromatic Phe84 on one side and Leu6 and Val9 on the opposite side, with the Trp149 indole donating a hydrogen bond ( Fig. 5 ). 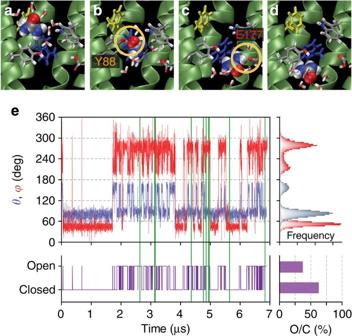Figure 5: Trp153 controls conduction through the cytoplasmic constriction. (a) Hydrated urea approaching the constriction from the periplasmic side. (b) Hydrogen bonding of the urea C=O with the Tyr88 O-H. (c) Hydrogen bonding of a urea N-H with the carboxyl C=O of Glu177. (d) Water breaks up this configuration (E), releasing the urea into the periplasmic vestibule. (e). Time evolution of the aromatic ring rotation angle of Trp153 for the 7-μs monomer simulation, showing that long timescales are essential for proper convergence. Spherical coordinatesθ(blue) andϕ(red) describe the aromatic plane configuration in the channel, which is open only if bothθ≈90° andϕ>180° (Supplementary Fig. S20). The analysis shows that the channel is closed for conduction ~63% of the time. Conduction events are indicated in green. Figure 5: Trp153 controls conduction through the cytoplasmic constriction. ( a ) Hydrated urea approaching the constriction from the periplasmic side. ( b ) Hydrogen bonding of the urea C=O with the Tyr88 O-H. ( c ) Hydrogen bonding of a urea N-H with the carboxyl C=O of Glu177. ( d ) Water breaks up this configuration (E), releasing the urea into the periplasmic vestibule. ( e ). Time evolution of the aromatic ring rotation angle of Trp153 for the 7-μs monomer simulation, showing that long timescales are essential for proper convergence. Spherical coordinates θ (blue) and ϕ (red) describe the aromatic plane configuration in the channel, which is open only if both θ ≈90° and ϕ >180° ( Supplementary Fig. S20 ). The analysis shows that the channel is closed for conduction ~63% of the time. Conduction events are indicated in green. Full size image Unlike for C P , no structural rearrangement was observed for C C over the course of the simulations (see Supplementary Fig. S8 ). Instead, C C was found to open transiently via aromatic side chain rotation of Trp153 by 78±12° around χ 2 from a horizontal (in the plane of the bilayer) to a vertical position pointing ‘up’ towards the periplasm ( Fig. 5 ). This reorientation of Trp153 is periodic and occurs on the timescale of tens to hundreds of nanoseconds. During the 7-μs monomer simulation, 225 transitions were observed, with the closed configuration on average lasting <t> closed =38±118 ns, nearly twice as long as the open configuration (<t> open =22±33 ns) ( Fig. 5 ). C C has a higher free energy barrier than C P for urea, and passage requires sequential hydrogen bond formation and breakage with key conserved residues, suggesting that it forms the selectivity filter. During passage through C C , the urea carbonyl first receives a hydrogen bond from the hydroxyl of Tyr88, which is later lost during transport across the constriction. Immediately, on the other side of the barrier the side chain carbonyl of protonated Glu177 offers a readily available hydrogen bond acceptor for one urea amino group ( Fig. 5 ). The simulations reveal that the hydrogen bond from Tyr88 is required for guiding urea into and through C C , which explains why the Y88F mutant was found to be non-functional in oocytes [5] (see also Supplementary Discussion and Supplementary Fig. S11 ). Hydrogen bonding to Glu177 might be important for allowing urea to break its bond with Tyr88 and hop over the constriction barrier; this is supported by the observation that the E177Q mutant is also functional [5] . After passage through C C , water rapidly releases urea from the cytoplasmic vestibule to complete the urea transport process. Water transport The vestibules of the Hp UreI channels were initially empty, but rapidly filled with a large number of water molecules during equilibration. Over the course of the simulations, water hydrates all parts of the pore including the two constriction sites (see Fig. 6 ). Remarkably, protomers were found to efficiently conduct water at single-channel rates of 2.6±0.9 × 10 9 s −1 for the hexamer and 4.8±2.7 × 10 9 s −1 for the restrained monomer (see Fig. 6 ), approximately four orders of magnitude larger than the urea conduction rate. Periodic rotation of Trp153 frequently changes the cross section of the cytoplasmic constriction C C , modulating the rate water conduction through the channel (see Fig. 6 ). The average dwell time for a water molecule in transit through the channel is just Δt=0.77±0.05 ns, a little longer than the time between consecutive permeation events (Δ t ′=0.21±0.04 ns). Both values are independent of the direction of water flux. 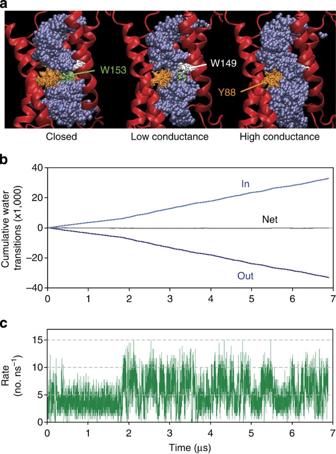Figure 6: Water flux through theHpUreI channel. (a) Water columns showing the open and closed states for water transport through aHpUreI protomer. The ‘open’ states (right panels) consist of continuous water channels and differ only in the width at the cytoplasmic constriction CC. The seal of the closed state is formed by Tyr88 and Trp153, with the latter acting as the gating residue. (b) A plot of the cumulative water transitions shows that the channel has no net water conduction. The average rate of water transport from fitting to the dotted lines is 4.8±0.6 water molecules per nanosecond per channel (both up and down). This is approximately four orders of magnitude higher than the rate of urea transport. (c) The water conduction rate (up and down, 2 ns average) as a function of time reveals that the channel is open to water ~99% of the time and has two conductance states. Low conduction (~3.5 × 109s−1) corresponds to a CCpartially closed by Trp153 (~62% of the time), whereas high conductance (~8 × 109s−1) is the result of a wide water channel due to Trp153 in the ‘open’ configuration (~37% of the time). The transitions between low and high conducting states are visible as slight changes in the slope for both upward and downward conduction (b). Figure 6: Water flux through the Hp UreI channel. ( a ) Water columns showing the open and closed states for water transport through a Hp UreI protomer. The ‘open’ states (right panels) consist of continuous water channels and differ only in the width at the cytoplasmic constriction C C . The seal of the closed state is formed by Tyr88 and Trp153, with the latter acting as the gating residue. ( b ) A plot of the cumulative water transitions shows that the channel has no net water conduction. The average rate of water transport from fitting to the dotted lines is 4.8±0.6 water molecules per nanosecond per channel (both up and down). This is approximately four orders of magnitude higher than the rate of urea transport. ( c ) The water conduction rate (up and down, 2 ns average) as a function of time reveals that the channel is open to water ~99% of the time and has two conductance states. Low conduction (~3.5 × 10 9 s −1 ) corresponds to a C C partially closed by Trp153 (~62% of the time), whereas high conductance (~8 × 10 9 s −1 ) is the result of a wide water channel due to Trp153 in the ‘open’ configuration (~37% of the time). The transitions between low and high conducting states are visible as slight changes in the slope for both upward and downward conduction ( b ). Full size image Water transport with similar single-channel rates (10 8 -10 9 s −1 ) has been observed for aquaporins [18] , [19] and voltage-gated sodium channels [17] . Conductance is equal in both directions, resulting in a zero net water transport through the channel pore in the absence of an osmotic gradient. While some UTs, such as the mammalian UT-B and the bacterial Ap UT, have been reported to conduct water [20] , [21] , UT-A has been shown not to conduct water [22] . This suggests that, although hydration of urea does not seem to be essential for urea transport per se , it might be important for urea transport through the Hp UreI channels. Although water flux through the channel is high, any significant conduction of protons through Hp UreI would almost certainly be lethal to H. pylori . During all simulations, Na and Cl ions (each at 100 mM concentration) generally do not enter the Hp UreI channel. The only exception is a single chloride ion in the 7-μs monomer simulation that briefly enters the cytoplasmic vestibule for ~2 ns before exiting again ( Supplementary Fig. S12 ). Analysis of the channel reveals that 63% of the channel-lining residues in the cytoplasmic vestibule are charged or polar compared with just 29% in the periplasmic vestibule ( Supplementary Fig. S13 ). A polar cytoplasmic vestibule probably serves to prevent urea moving backwards through the channel after having traversed C C , while the hydrophobic lining of the periplasmic vestibule almost certainly serves to discourage ions to enter the channel. Sodium ions generally enter much deeper into the bilayer than Cl − , due to hydrogen bonding interactions with the phosphate head groups, which are located closer to the core of the bilayer [23] , [24] , [25] . Nevertheless, Na + avoids the full length (~20 Å) of the channel pore ( Supplementary Fig. S12 ). Similarly, NH 4 + (at 75 mM concentration) also does not enter the channel ( Supplementary Fig. S14 ). These findings suggest that the periplasmic vestibule and constrictions are too hydrophobic to allow ions to pass through the channel. Conduction of NH 3 and CO 2 The 2NH 3 and 1CO 2 produced for each urea hydrolyzed in the cytoplasm need to reach the periplasm before picking up a proton (NH 3 to NH 4 + ) or being converted to carbonic acid (CO 2 to H 2 CO 3 to H + +HCO 3 − ), the latter being catalysed by a periplasmic carbonic anhydrase ( Supplementary Fig. S1 ) [26] . To check the retrograde pathway of the hydrolysis products, we performed equilibrium simulations in the presence of NH 3 and CO 2 . Both solutes were found to preferentially go through the bulk bilayer and the central lipid plug, and the rate in both cases is much higher than the urea flux rate, suggesting no particular molecular mechanism is required to provide efficient efflux of buffering products to the periplasm. The permeation rate for CO 2 is 4.5 × 10 6 s −1 at 5 mM concentration, while the rate for NH 3 is 2.0 × 10 6 s −1 at 10 mM concentration ( Supplementary Fig. S15 ). This result agrees with previous molecular dynamics simulations that demonstrated that both CO 2 and NH 3 can easily cross membranes of different compositions and do not require specific proteins for transport [27] . Unbiased microsecond equilibrium molecular dynamics simulations of Hp UreI have been used to study the mechanism of urea conduction at atomic detail (see Fig. 1 ). The hexameric assembly was found to be critical to preserve the structural integrity of the channels in the membrane ( Supplementary Fig. S2 ). This unusual arrangement might serve to ensure a tight seal between Hp UreI and the cytoplasmic urease to avoid toxic alkalinization of the cytoplasm by the NH 3 produced by urea hydrolysis ( Supplementary Fig. S16 ). The arrangement might also play a role in the pH gating of the channel by periplasmic loop folding cooperatively or onto neighboring channels. Hp UreI is selective for urea and closely related molecules [5] , [8] , [28] , but nevertheless has a remarkably low binding affinity for urea (K d =~163 mM) [8] , and no ordered urea was observed in the crystal structure [5] . The simulations reveal that this low affinity is due to a combination of dehydration and confinement of urea in the Hp UreI channel. Water molecules lost from the bulk water hydration shell cannot be fully replaced by contacts with pore-lining side chains because of a lack of sufficient hydrogen bonding partners, resulting in an energetic penalty associated with urea dehydration. In addition, the simulations show that urea, which has a liquid state dipole moment of 6–8 D [11] , preferentially orients inside the channel during transport, with the amino groups pointing away from the central lipid plug (see Fig. 2 ), resulting in an energetic penalty associated with a reduction in entropy. The net alignment of urea in the channel, observed in the simulations, matches the electrostatic charge distribution on the periplasmic channel surface, previously derived by electrostatic potential calculations [5] , with the carbonyl group pointing towards a positive protein surface facing the central plug and the amino groups facing towards a negative protein surface directed towards the bulk lipids in the bilayer. The surface charge arrangement might serve to correctly pre-orient urea molecules for efficient transport through the selectivity filter further inside the channel pore. A total of 15 urea transport events were captured in the simulations of wild-type Hp UreI. Scaled to 5 mM, which is much closer to the gastric urea concentration, this corresponds to a single-channel conduction rate of 10 3 –10 4 s −1 . This value seemed low, given that channel proteins usually display solute transport rates that are several orders of magnitude higher, achieving single-pore permeation rates of 10 6 –10 9 s −1 (refs 15 , 17 ). This result prompted us to experimentally determine the urea conduction rates in H. pylori cells [5] , giving an approximately single-channel transport rate of 10 2 –10 3 s −1 , which is lower than the rate of ~10 4 s −1 , derived from previous measurements of urea flux through Hp UreI channels in proteoliposomes [8] . Nevertheless, both experimental and simulation results confirm that the urea conduction rate is much lower than that of typical channel proteins. One reason might be that high conducting channels typically conduct smaller entities, such as water or monatomic ions. Indeed, the rate of water transport through Hp UreI was found to be much higher, equivalent to that of aquaporins (see below). For the structurally completely unrelated mammalian urea transporters, single-channel rates of 10 4 s −1 have been recorded in the presence of a 500 mM urea gradient [29] , which corresponds to a rate of ~10 2 s −1 at 5 mM. This suggests that Hp UreI is a much more efficient channel at low urea concentration gradients, which may be one explanation why H. pylori uses this particular channel for uptake of gastric urea, rather than a UT channel homologue, which also occur in bacteria, presumably for nitrogen nutrient uptake [30] . Another explanation might be that UTs generally do not show pH gating, essential for H. pylori ’s urea channel, although this might have well developed evolutionary, just as some UreI homologues do not show pH gating. Both UT and Hp UreI channels have similar half-saturation urea concentrations of over 100 mM [8] , [21] , [31] , [32] . The Hp UreI crystal structure revealed two constrictions in the channel, which open transiently during the simulations to allow passage of urea. 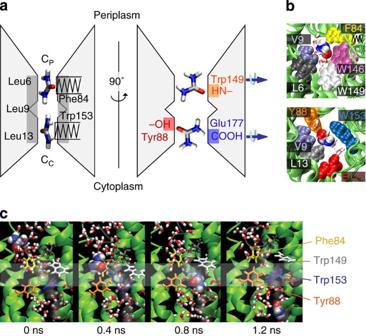Figure 7: Urea transport mechanism. (a): Schematic of the urea conduction mechanism ofHpUreI. During transport through the adjacent constriction sites CP(periplasmic) and CC(cytoplasmic), urea is sandwiched between highly conserved residues, while simultaneously hydrogen bonding to orthogonally oriented sidechains. CPis much more hydrophobic, probably to reject protons, while CCselects for urea-like molecules. Although the channel architecture is completely different, a somewhat analogous local arrangement was observed in the UT channels, where urea was found to be sandwiched between two Phe sidechains with a Glu residue accepting hydrogen bonds from the urea amino groups6. (b) Aromatic residues (Phe84, Trp153) wedge urea against a wall of hydrophobic residues (Leu6, Val9, and Leu13), while orthogonal residues W149 and Tyr88 present hydrogen bonding groups and prevent complete desolvation of the constriction sites. (c) Spontaneous urea transport through the central constriction (site 2, shaded grey) of a channel protomer, which obstructs the pore of the water-filled channel in the crystal structure. Rotation of the indole moiety of Trp153 towards the periplasm through rotation around χ2transiently opens the constriction allowing the passage of urea (two central panels). The constriction closes again shortly afterwards with the Trp153 orientation returning to that observed in the crystal structure. Even in their open states, the constrictions remain largely hydrophobic and narrow ( Figure 7 ). The free energy profile along the channel pore, which was determined from the urea number density in the pore at equilibrium (see Methods ), shows that the periplasmic constriction C P has a barrier for urea transport of ~2 kcal mol −1 , significantly lower than the ~3.5 kcal mol −1 barrier observed for C C ( Fig. 2 ). Together with the observation that the C P is more hydrophobic (that is, offers less hydrogen bonding partners) than C C, this suggests that C P and C C probably function as proton rejection and urea selectivity filters, respectively. Figure 7: Urea transport mechanism. ( a ): Schematic of the urea conduction mechanism of Hp UreI. During transport through the adjacent constriction sites C P (periplasmic) and C C (cytoplasmic), urea is sandwiched between highly conserved residues, while simultaneously hydrogen bonding to orthogonally oriented sidechains. C P is much more hydrophobic, probably to reject protons, while C C selects for urea-like molecules. Although the channel architecture is completely different, a somewhat analogous local arrangement was observed in the UT channels, where urea was found to be sandwiched between two Phe sidechains with a Glu residue accepting hydrogen bonds from the urea amino groups [6] . ( b ) Aromatic residues (Phe84, Trp153) wedge urea against a wall of hydrophobic residues (Leu6, Val9, and Leu13), while orthogonal residues W149 and Tyr88 present hydrogen bonding groups and prevent complete desolvation of the constriction sites. ( c ) Spontaneous urea transport through the central constriction (site 2, shaded grey) of a channel protomer, which obstructs the pore of the water-filled channel in the crystal structure. Rotation of the indole moiety of Trp153 towards the periplasm through rotation around χ 2 transiently opens the constriction allowing the passage of urea (two central panels). The constriction closes again shortly afterwards with the Trp153 orientation returning to that observed in the crystal structure. Full size image A significantly higher barrier of ~5.0 kcal mol −1 was obtained from potential-of-mean-force (PMF) calculations of a non-homologous UT channel [7] , which is consistent with a lower conduction rate of UT compared with Hp UreI channels at low urea concentrations. Although UTs possess an entirely different architecture compared with Hp UreI, the free energy profile for transport of urea through the pore is similar, with two closely spaced barriers near the center of each channel ( Fig. 2 ) [7] . The UT profile is at least partly due to the two-fold pseudo symmetry of the long, narrow UT pore, explaining the equal height of both barriers. Hp UreI displays no such symmetry. While both the Hp UreI and UT free energy profiles are primarily the result of the cost of urea desolvation in the channel, the level of hydration is very different. In the Hp UreI channel urea is always hydrated by at least four water molecules, while the maximum observed in the UT channel was less than three [7] . This explains why UT channels have higher transport barriers. Several aquaglyceroporins, which can carry a range of solutes other than water across membranes, also conduct urea. For these proteins, the size of the pore, in particular at the aromatic/arginine (ar/R) constriction, seems to be the major factor determining urea conduction [33] , [34] , [35] . Indeed, widening the ar/R constriction by mutating bulky aromatics to small residues in a water-specific aquaporin (AQP1) enabled efficient conduction of urea and glycerol, without affecting water permeability [36] . This suggests that sufficient space and a high level of hydration are key requirements for urea conduction, irrespective of the pore chemistry. The simulations identify a sequential interaction of urea with highly conserved residues that determine selectivity and control urea flux through the channel and are located at the cytoplasmic constriction C C . In particular, urea selectivity by Hp UreI depends critically on χ 2 rotation of the indole moiety of Trp153, which opens the closed cytoplasmic constriction observed in the crystal structure for spontaneous conduction ( Fig. 4 ). These rotations are transient and occur on the timescale of tens to hundreds of nanoseconds, necessitating microsecond simulations. In the open configuration, Trp153 acts as a lever that pins urea against a hydrophobic wall formed by the highly conserved residues Leu6, Val9, and Leu13 ( Fig. 7 & Supplementary Fig. S17 ), suggesting that this constriction forms the selectivity filter for planar urea-like molecules. This finding explains why both W153A and W153F mutants showed decreased selectivity for urea, while the overall urea transport rate for these mutants was similar to that of wild type [5] . While Trp153 is vital for selectivity and for maintaining an open pore configuration, hydrogen bonding interactions of urea with the hydroxyl group of Tyr88 are essential for guiding urea through the cytoplasmic constriction ( Fig. 7 ). This finding explains why the experimental Y88F mutant does not conduct urea [5] . Although the overall channel architecture is entirely unrelated, a striking similarity between Hp UreI and both bacterial and mammalian UT channels is the prominent arrangement of combinations of aromatic and hydrophobic residues in the pore [6] . For both channel types, urea has to pass through the pore sandwiched between either a pair of aromatic residues or an aromatic and hydrophobic residues, with other residues offering hydrogen bonding groups (see Fig. 7 ) [5] , [7] , presumably to ensure high selectivity for a planar urea molecule that is also highly polar. Amide-π stacking interactions have been suggested to aid stabilization of this configuration [6] , [37] . While both UT and Hp UreI channels use this aromatic sandwiching motif, the proposed mechanism of urea transport differs. Hp UreI features an hourglass shaped channel pore lined exclusively with flexible side chains, only half of which are capable of forming hydrogen bonds with urea. Most of the hydrogen bonding in the channel pore, even at the constriction sites, is provided by water molecules that solvate the entire Hp UreI channel pore during conduction ( Fig. 6 ). In contrast, UTs have cylindrical pores that are narrow along their entire length and cannot provide the same level of aqueous hydration [7] , but are instead lined by a continuous ladder of hydrogen bond acceptors provided by the polypeptide backbone carbonyl oxygens, which are presumed to guide urea through the UT channel pore [6] , [7] . Furthermore, based on the location of dimethylurea and selenourea in the crystal structures of Dv UT and UT-B, respectively, UT pores have been proposed to contain two low affinity urea binding sites, which allow multiple coordination with the urea carbonyl and amino groups, reflected in the low dissociation constant ( K d =2.3±0.1 mM) [6] , [7] . No binding sites are observed in Hp UreI, which has a much lower affinity for urea ( K d =~163 mM) [8] ( Fig. 2 ). Remarkably, the simulations revealed that Hp UreI conducts water at a single-channel rate of ~10 9 s −1 , which is similar to the rate of aquaporins [18] , [19] . While the cytoplasmic constriction C C is able to shut the channel to water transport completely, this occurs for only ~1% of the time. The pore chiefly alternates between partially and fully open states, which show a continuous water column that connects the periplasmic with the cytoplasmic vestibules (see Fig. 6 ). This raises the question how Hp UreI prevents the flux of protons along a Grotthus proton wire through the channel pore. Recent studies on aquaporins have shown that the large free energy penalty associated with ionic desolvation inside a narrow hydrophobic channel is sufficient to prevent proton conduction, even when a Grotthus proton wire can form [38] , [39] , which suggests that in Hp UreI the periplasmic constriction serves as the proton rejection filter. Furthermore, Na + , Cl − , and NH 4 + do not enter the periplasmic vestibule or the constrictions during the simulations, demonstrating that this part of the pore is sufficiently narrow and hydrophobic to block hydrated ions ( Supplementary Figs S12 and S14 ). Compared with UTs, some of which have also been reported to conduct water [21] , Hp UreI has a wider pore that allows a much larger number of water contacts (see Fig. 2 ). This reduces the urea desolvation penalty in the channel and lowers the barrier height for transport, suggesting that efficient conduction of urea at low concentrations, which is essential to the survival of H. pylori , might rely on increased urea hydration during transport. Long timescale unbiased equilibrium molecular dynamics simulations were employed to investigate the mechanism of urea conduction of Hp UreI at atomic detail. The computational effort for this study was considerable, with cumulative simulation times of over 10 μs for the Hp UreI monomer and over 3 μs for the hexameric channel assembly. These simulations took over 1 year to complete, using some of the world’s fastest high performance clusters, including the Anton supercomputer at the Pittsburg Supercomputing Center, which has hardware specifically designed for efficient molecular dynamics simulations [40] . Although the computational effort is 1–2 orders of magnitude larger than for steered or biased simulations (for example, potentials of mean force derived by umbrella sampling), the advantage of equilibrium simulations is that they reveal a great wealth of atomic resolution mechanistic, thermodynamic, and kinetic details that cannot be obtained by any other approach. In the present study, the simulations reveal how the closed pore of the crystal structure of Hp UreI opens to allow conduction of urea and identify the proton rejection and selectivity roles of the two central constrictions in the channel. Aromatic ring rotations with periodicities of tens to hundreds of nanoseconds were found to alternate the conduction properties of the channel, requiring sufficiently long simulation timescales to derive urea conduction rate estimates. The simulations reveal that the channel conducts water at high rates while rejecting ions. This demonstrates that with sufficient computational resources long-timescale equilibrium simulations are an excellent tool to complement structural and physiological experimental techniques, providing high-quality information on atomic detail mechanisms. Model building The hexameric Hp UreI channel arrangement from the crystal structure (PDB code 3UX4) was used as the starting structure. Periplasmic loop 1 (PL1) between residues 59–72 was not resolved in the crystal structure. These residues were modelled as an extended loop onto a single protomer using the program hippo beta ( www.biowerkzeug.com ). Missing atoms were added using hippo beta, and the protomer was inserted into a palmitoyloleoyl-phosphocholine (POPC) lipid bilayer and equilibrated for 400 ns, while restraining the protein atoms to the crystal structure coordinates. PL1 showed considerable flexibility ( Supplementary Fig. S18 ). The equilibrated modelled loop from the monomer simulation was copied and transposed onto the Hp UreI hexamer crystal structure. Lipids in the central plug were modelled to match the number of fatty acid tails resolved in the crystal structure (that is, three POPC lipids to match the six fatty acid tails in the narrower periplasmic leaflet of the plug and nine POPC lipids matching the 18 fatty acid tails in the wider cytoplasmic leaflet). The system was equilibrated for 50 ns at 37 °C with strong harmonic position restraints on the protein. Protonation states of ionizable residues depend on the pH of the system and the local pK a of the ionizable group. The crystal structure was determined at pH 5.3, and protonation states were chosen such that the periplasmic residues are at pH 5.3, while cytoplasmic pH was assumed to be 7.0. The protonation states are summarized in Supplementary Table S3 . Molecular dynamics simulations Molecular simulations were performed using GROMACS 4.5 ( www.gromacs.org ) [41] , with the OPLS all-atom protein force field [42] , the TIP3P water model [43] , and OPLS united-atom lipid parameters for POPC [44] . Additional simulations were performed using the Anton supercomputer at the Pittsburgh Supercomputing Center, with the CHARMM27 protein [45] and CHARMM36 lipid force fields [46] , and TIP3P water models (3). Initial configurations for the Anton runs were created using DESMOND software [40] . All simulations were analysed using hippo beta ( www.biowerkzeug.com ). Electrostatic interactions were computed using the particle mesh Ewald (PME) method [47] , and a cutoff of 10 Å was used for van der Waals interactions. Bonds involving hydrogen atoms were restrained using LINCS [48] . Simulations were run with a 2 fs integration time step, and neighbour lists were updated every five steps. All simulations are performed in the NPT ensemble, with no additional applied surface tension. Solvent (water, ions, and urea), lipids and the protein were each coupled separately to a heat bath at a temperature of 37 °C with time constant τ T =0.1 ps using weak temperature coupling [49] . Atmospheric pressure of 1 bar was maintained using weak semi-isotropic pressure coupling with compressibility κ z =κ xy =4.6·10 –5 bar –1 and time constant τ P =1 ps [50] . Hexameric simulations were performed without any restraints, while simulations of monomeric protomers were performed both with and without harmonic backbone restraints on the protein. A complete list of simulations is given in Supplementary Table S1 . Free energy profiles Transmembrane solute free energy profiles were calculated from the occupancy of urea in the channel pore as a function of centre of mass position along the membrane normal. For a system in thermodynamic equilibrium, the occupancy of states is related to the free energy by where R is the ideal gas constant, T is the temperature, and f (z) is the normalized occupancy of solutes at z . The relative free energy was calculated for each bin, and the minimum was shifted to zero. Potential of mean force (PMF) calculations To estimate the barrier of various compounds in the channel, PMF calculations were performed on a UreI monomer embedded in a POPC bilayer for urea, thiourea, and H 3 O + . The reaction coordinate was taken from the first spontaneous transport event. Evenly spaced windows 0.5 Å apart were selected manually. For each window a 5-ns simulation was performed to obtain the free energy profile along the channel pathway using the weighted histogram analysis method (WHAM) [51] . For these simulations, the monomeric simulation system was used and protein backbone atoms were position restrained with harmonic potentials to ensure the protein remains close to the native structure. The PMF trans-bilayer free energy profile was also calculated for urea crossing a POPC lipid bilayer ( Supplementary Fig. S19 ). The 0.5 Å spacing and 5 ns timescales at each window proved inadequate to produce converged PMF profiles, and the results were not included in this study (see Supplementary Table S4 ). This is most likely due to the fact that the channel pore is lined exclusively by side chains, which need much longer sampling times to explore all rotameric states accessible at equilibrium. This applies particularly to the conserved aromatic chains of the constrictions that have reorientation timescales of tens to hundreds of nanoseconds ( Figs 4 and 5 ). How to cite this article: McNulty, R. et al. Mechanisms of molecular transport through the urea channel of Helicobacter pylori . Nat. Commun. 4:2900 doi: 10.1038/ncomms3900 (2013).